JAK/STAT3 signalling is sufficient and dominant over antagonistic cues for the establishment of naive pluripotency Induced pluripotency depends on cooperativity between expression of defined factors and the culture environment. The latter also determines the pluripotent cell state, that is, naïve or primed. LIF-JAK/STAT3 signalling was recently shown to be a limiting factor for reprogramming to naïve pluripotency. Here we show that sufficient activation of JAK/STAT3 overcomes the reprogramming block of cell intermediates and enables somatic cell reprogramming in absence of otherwise essential pluripotency medium requisites. Activation of FGF-ERK signalling, which promotes exit of naïve pluripotent cells from self-renewal, does not prevent JAK/STAT3 induced post-implantation epiblast-derived stem cell conversion into naïve pluripotency. Moreover, even in the presence of FGF plus Activin, which instructs and maintains the primed state, JAK/STAT3 enforces naïve pluripotency in epiblast stem cells. We conclude that JAK/STAT3 signalling can be sufficient and dominant over antagonistic cues to enable the induction of a naïve pluripotent state. Pluripotency can be reinstated into somatic cells by expression of defined transcription factors [1] . During this process, cells are maintained in culture conditions that support self-renewal of pluripotent cells. Importantly, it has become apparent that the culture environment is also actively involved in the reprogramming process and is a key determinant for the outcome of the pluripotent cell state, that is, naïve or primed pluripotency. Wnt signalling and inhibition of MEK/ERK signalling were shown to promote induction of somatic cells to an embryonic stem (ES) cell like state, which is defined as naïve pluripotency [2] , [3] , [4] . This cell state has similar functional properties to the pre-implantation epiblast as on introduction in the blastocyst cells enter embryonic development and contribute to the adult animal. On the other hand, FGF and Activin signalling promote reprogramming of somatic cells to a pluripotent cell state that is characteristic of post-implantation epiblast-derived stem cells (EpiSCs) and which is described as primed pluripotency [5] , [6] , [7] . Primed and naïve pluripotent cells share some core transcriptional regulators but are clearly distinct from each other in aspects including epigenetic status, developmental capacity and culture requirements [2] . Recently, it was found that activation of JAK/STAT3 is a limiting component for the induction of naïve pluripotency [8] . This was demonstrated by both its ability to enhance somatic cell reprogramming efficiency and to reprogramme EpiSCs to naïve pluripotency. In ES cells, JAK/STAT3 signalling is activated by leukaemia inhibitory factor (LIF). LIF plus serum defines the classic culture environment that enables the infinite self-renewal of ES cells [9] , [10] . LIF contributes to this via the LIFRβ-GP130 signal transducer receptor complex that activates JAK kinases, which then phosphorylate latent transcription factor STAT3 (refs 11 , 12 ). On phosphorylation STAT3 dimerizes and enters the nucleus to regulate transcription. Recently, we reported that overexpression of Nanog enables somatic cell reprogramming in minimal culture conditions [13] . However, this required the presence of LIF in the medium. Derived Nanog-iPS cells did not require LIF for self-renewal indicating that the critical role of LIF in this context resided in the acquisition, but not maintenance, of pluripotency. Here we assessed the capacity of JAK/STAT3 for the reprogramming of cells towards a naïve pluripotent state in different cell contexts and culture conditions. This revealed that JAK/STAT3 is sufficient to enable reprogramming in the absence of additional pluripotency culture requisites and dominantly enforces naïve pluripotency in a culture environment that instructs and maintains a primed cell state. Elevated JAK/STAT3 overcomes the pre-iPS reprogramming block Mouse somatic cells transduced with retroviruses containing the canonical reprogramming factors and cultured in serum plus LIF medium frequently fail to complete reprogramming [4] , [14] . These cells become trapped in a proliferative cell state and were named pre-iPS cells as full induction of pluripotency proceeds only on medium switch to one containing inhibitors of the MEK/ERK signalling pathway or DNA methylation [4] , [13] , [14] . As JAK/STAT3 signalling has been identified as a limiting component in the reprogramming process, we investigated whether increased activation of this pathway could also overcome the pre-iPS cell reprogramming block observed in serum plus LIF culture conditions. To activate JAK/STAT3, we used the granulocyte colony-stimulating factor (G-CSF) inducible GY118F chimaeric LIF receptor transgene. This is a fusion protein constituted of the external ligand-binding domain of the G-CSF receptor and the transmembrane and cytoplasmatic GP130 signal-transducing domain of the LIF receptor. In addition, the cytoplasmic GP130 domain contains a mutation that causes an amino-acid substitution at residue 118 from tyrosine to phenylalanine. This leads to specific activation of the JAK-STAT3 pathway, leaving RAS-MAPK and PI3 kinase unactivated [15] . This mutation also interferes with binding of the negative feedback regulator Socs3, resulting in elevated and sustained STAT3 signalling [16] , [17] . The GY118F transgene or empty vector were transfected into a stable clonal pre-iPS cell line generated from female mouse embryonic fibroblasts (MEFs). These cells contain a GFP reporter driven by Oct4 regulatory sequences (Oct4-GFP). Stimulation of stably transfected GY118F pre-iPS cells with G-CSF resulted in the phosphorylation of STAT3 and transcriptional activation of its direct target Socs3 ( Fig. 1a ). After one week in the presence of G-CSF Oct4-GFP-positive colonies were found in GY118F-transfected cells, but not in controls ( Fig. 1b ). Flow cytometry analysis revealed an increasing proportion of Oct4-GFP expressing cells that comprised 3.0% at day 7 and 11.8% at day 13 on addition of G-CSF ( Fig. 1c ). Low level Oct4-GFP expressing cells were detected in controls but, as previously shown, this corresponded to unstable non-pluripotent reporter expression [13] . GY118F Oct4-GFP-positive cells were isolated by flow cytometry ( Fig. 1d ) and subsequently analysed for their pluripotent status. These cells expressed pluripotency-associated genes and silenced the retroviral transgenes ( Fig. 1e ). They also reactivated the silent X-chromosome as indicated by the loss of both the trimethyl(me3)H3K27 nuclear body [18] ( Fig. 1f ) and the Xist RNA cloud ( Fig. 1g ). Additionally, the appearance of Xist RNA pinpoint signals, corresponding to the detection of nascent transcripts from the two Xist alleles, is indicative of reprogramming to naive pluripotency [19] . One mechanism by which the pre-iPS cell serum reprogramming block can also be overcome is by inhibition of the MEK/ERK signalling pathway [4] . However, western blot analysis showed no apparent change in phospho-ERK levels, the active form of ERK, in G-CSF stimulated GY118F pre-iPS cells ( Fig. 1h ), suggesting that JAK/STAT3 overcomes the pre-iPS cell reprogramming block by an alternative mechanism. Together, these results show that increased activation of JAK/STAT3 has the capacity to overcome reprogramming barriers. 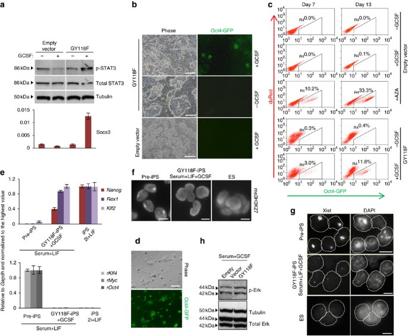Figure 1: Increased activation of JAK/STAT3 overcomes the pre-iPS cell reprogramming block. (a) phospho (p) -STAT3 western blot andSocs3quantitative real-time PCR (qRT–PCR) demonstrating activation of GY118F by G-CSF in pre-iPS cells. Pre-iPS cells harbouring an empty vector were used as a control. Error bars indicate ±1 s.d. (n=3). (b–g) Reprogramming of female GY118F pre-iPS cells in serum and LIF culture conditions and subsequent analysis. (b) Appearance of GFP-positive colonies indicates activation of the Oct4 reporter transgene. White bars correspond to 178.8 μm. (c) Flow cytometry analysis of GY118F pre-iPS cells at day 7 and day 13 after addition of G-CSF. The percentage of Oct4-GFP-positive cells is indicated above the gate. Pre-iPS cells harbouring an empty vector were used as a control. 5-Azacytidine was used as a positive control for the reprogramming of pre-iPS cells. (d) Phase and fluorescent images of isolated GY118F Oct4-GFP-positive cells in serum plus LIF plus G-CSF. The white bar corresponds to 161 μm. (e) qRT–PCR analysis for pluripotency marker genes and retroviral (r) transgenes. iPS cells cultured in 2i plus LIF medium were used as a control. Gene expression and associated error bars representing s.d. (n=3) were normalized to the sample with highest expression. (f) Immunofluorescence for trimethyl(me3)H3K27 of GY118F iPS cells. Parental pre-iPS cells and female ES cells were used as controls. White bars correspond to 14.5 μm. (g) Fluorescentin situhybridizations (FISH) for Xist RNA on GY118F iPS cells. Parental pre-iPS cells were used as a control for the presence of the inactive X chromosome. Male ES cells were used as a positive control for Xist pinpoint signal. White dashed lines outline examples of individual cell nuclei. White bars correspond to 8.8 μm. (h) Western blot analysis for phospho-ERK of GY118F or control vector pre-iPS cells stimulated with G-CSF for 24 h. Tubulin and total ERK were used as loading controls. Figure 1: Increased activation of JAK/STAT3 overcomes the pre-iPS cell reprogramming block. ( a ) phospho (p) -STAT3 western blot and Socs3 quantitative real-time PCR (qRT–PCR) demonstrating activation of GY118F by G-CSF in pre-iPS cells. Pre-iPS cells harbouring an empty vector were used as a control. Error bars indicate ±1 s.d. ( n =3). ( b – g ) Reprogramming of female GY118F pre-iPS cells in serum and LIF culture conditions and subsequent analysis. ( b ) Appearance of GFP-positive colonies indicates activation of the Oct4 reporter transgene. White bars correspond to 178.8 μm. ( c ) Flow cytometry analysis of GY118F pre-iPS cells at day 7 and day 13 after addition of G-CSF. The percentage of Oct4-GFP-positive cells is indicated above the gate. Pre-iPS cells harbouring an empty vector were used as a control. 5-Azacytidine was used as a positive control for the reprogramming of pre-iPS cells. ( d ) Phase and fluorescent images of isolated GY118F Oct4-GFP-positive cells in serum plus LIF plus G-CSF. The white bar corresponds to 161 μm. ( e ) qRT–PCR analysis for pluripotency marker genes and retroviral (r) transgenes. iPS cells cultured in 2i plus LIF medium were used as a control. Gene expression and associated error bars representing s.d. ( n =3) were normalized to the sample with highest expression. ( f ) Immunofluorescence for trimethyl(me3)H3K27 of GY118F iPS cells. Parental pre-iPS cells and female ES cells were used as controls. White bars correspond to 14.5 μm. ( g ) Fluorescent in situ hybridizations (FISH) for Xist RNA on GY118F iPS cells. Parental pre-iPS cells were used as a control for the presence of the inactive X chromosome. Male ES cells were used as a positive control for Xist pinpoint signal. White dashed lines outline examples of individual cell nuclei. White bars correspond to 8.8 μm. ( h ) Western blot analysis for phospho-ERK of GY118F or control vector pre-iPS cells stimulated with G-CSF for 24 h. Tubulin and total ERK were used as loading controls. Full size image JAK/STAT3 signalling is sufficient to enable reprogramming The results described above, together with the previous finding that activation of JAK/STAT3 enhances reprogramming efficiency [8] argues for a potent role in instructing naïve pluripotency. Therefore, we asked whether increased activation of JAK/STAT3 could enable somatic cell reprogramming in a culture environment where no additional ES cell self-renewal factors are present. To address this, we used basal N2B27 medium. This is a defined serum-free medium that to support the induction and maintenance of naïve pluripotency must contain two or more additional culture environment factors, that is, feeder cells, LIF, BMP4, MEK/ERK- and GSK3- kinase inhibitors [20] , [21] . Female adult neural stem (aNS) cells, containing an Oct4-GFP reporter, were stably transfected with the GY118F transgene or empty vector. Addition of G-CSF to GY118F aNS cells rapidly led to the upregulation of Socs3 , a direct target of STAT3 ( Fig. 2a ). GY118F or control aNS cells were transduced with retroviral Oct4, Klf4 and c-Myc. Following infection, the cells were cultured in NS cell medium for 5 days and then in N2B27 with or without G-CSF. In contrast to controls, G-CSF-stimulated GY118F plates showed Oct4-GFP-positive colonies after 10 days ( Fig. 2b ). Oct4-GFP-positive cells were isolated by flow cytometry and maintained in N2B27 plus G-CSF medium ( Fig. 2c ). These cells exhibited the profile of a naïve pluripotent state, as shown by the activation of pluripotency genes, silencing of retroviral transgene expression ( Fig. 2d ) and loss of both the me3H3K27 nuclear body ( Fig. 2e ) and Xist RNA cloud ( Fig. 2f ). To assess the reprogramming efficiency in terms of iPS cell colony generation, we replated 6×10 4 transduced GY118F aNS cells in N2B27 with or without G-CSF. After 12 days, 47±11 ( n =3) Oct4-GFP-positive colonies were observed in G-CSF-treated cells as opposed to none in untreated cells. Control iPS and ES cells cannot self-renew in N2B27 plus LIF or N2B27 with or without G-CSF ( Supplementary Fig. S1a ). In agreement with this on withdrawal of G-CSF GY118F iPS cells lost Oct4-GFP reporter activity and differentiated ( Fig. 2g,h ). GY118F iPS cells could also grow interchangeably in medium containing inhibitors for MEK/ERK and GSK3 (2i), a culture condition that is both supportive and selective for naïve pluripotent cells ( Supplementary Fig. S1b ). On blastocyst injection GY118F iPS cells, derived and maintained in N2B27 plus G-CSF, showed contribution to the adult animal confirming their pluripotent nature ( Fig. 2i ). 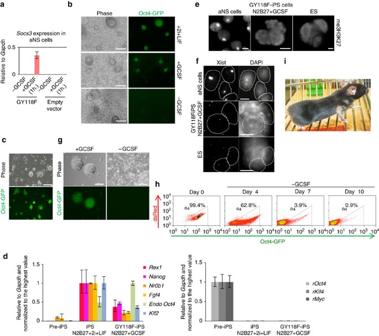Figure 2: Sufficient JAK/STAT3 activation eliminates the need for pluripotency culture requisites in somatic cell reprogramming. (a) Female aNS cells containing the GY118F transgene showing activation of direct STAT3 targetSocs3on stimulation with G-CSF for 1 h. Error bars indicate ±1 s.d. (n=3). (b,c) Reprogramming of aNS cells. The cells were infected with retroviral Oct4, Klf4 and c-Myc and subsequently stimulated with G-CSF in N2B27 medium only. (b) GFP expression indicates activation of the Oct4 reporter transgene. N2B27 plus 2i plus LIF medium was used as a positive control for reprogramming. White bars correspond to 195 μm. (c) Phase and fluorescent images depicting the derived GY118F iPS cells maintained in N2B27 plus G-CSF. The white bar corresponds to 182.6 μm. (d–i) Analyses of the GY118F iPS cells derived and maintained in N2B27 plus G-CSF. (d) qRT–PCR analysis for pluripotency marker genes and retroviral (r) transgenes. iPS cells cultured in 2i plus LIF were used as a control. Endo, endogenous. Gene expression and associated error bars representing s.d. (n=3) were normalized to the sample with highest expression. (e) Immunostaining of GY118F iPS cells for me3H3K27. aNS cells show a me3H3K27 focus, unlike iPS or control female ES cells. White bars correspond to 6.4 μm. (f) FISH for Xist RNA on GY118F iPS cells. aNS cells and male ES cells were used as controls. White dashed lines outline examples of individual cell nuclei. White bars correspond to 8.8 μm. (g) Phase and fluorescence images of GY118F iPS cells after withdrawal of G-CSF from N2B27. White bars correspond to 184 μm. (h) Flow cytometry analysis for Oct4-GFP reporter expression after G-CSF withdrawal from GY118F iPS cell culture. Percentage is indicated above the gate. (i) Agouti coat colour reflects contribution of GY118F iPS cells on blastocyst injection. Figure 2: Sufficient JAK/STAT3 activation eliminates the need for pluripotency culture requisites in somatic cell reprogramming. ( a ) Female aNS cells containing the GY118F transgene showing activation of direct STAT3 target Socs3 on stimulation with G-CSF for 1 h. Error bars indicate ±1 s.d. ( n =3). ( b , c ) Reprogramming of aNS cells. The cells were infected with retroviral Oct4, Klf4 and c-Myc and subsequently stimulated with G-CSF in N2B27 medium only. ( b ) GFP expression indicates activation of the Oct4 reporter transgene. N2B27 plus 2i plus LIF medium was used as a positive control for reprogramming. White bars correspond to 195 μm. ( c ) Phase and fluorescent images depicting the derived GY118F iPS cells maintained in N2B27 plus G-CSF. The white bar corresponds to 182.6 μm. ( d – i ) Analyses of the GY118F iPS cells derived and maintained in N2B27 plus G-CSF. ( d ) qRT–PCR analysis for pluripotency marker genes and retroviral (r) transgenes. iPS cells cultured in 2i plus LIF were used as a control. Endo, endogenous. Gene expression and associated error bars representing s.d. ( n =3) were normalized to the sample with highest expression. ( e ) Immunostaining of GY118F iPS cells for me3H3K27. aNS cells show a me3H3K27 focus, unlike iPS or control female ES cells. White bars correspond to 6.4 μm. ( f ) FISH for Xist RNA on GY118F iPS cells. aNS cells and male ES cells were used as controls. White dashed lines outline examples of individual cell nuclei. White bars correspond to 8.8 μm. ( g ) Phase and fluorescence images of GY118F iPS cells after withdrawal of G-CSF from N2B27. White bars correspond to 184 μm. ( h ) Flow cytometry analysis for Oct4-GFP reporter expression after G-CSF withdrawal from GY118F iPS cell culture. Percentage is indicated above the gate. ( i ) Agouti coat colour reflects contribution of GY118F iPS cells on blastocyst injection. Full size image Recently, it was reported that ES cells overexpressing a mutant form of JAK2 (JAK2V617F) can self-renew in N2B27 only [22] . JAK2V617F is active without stimulation by cytokines and apparently confers this phenotype independently of STAT3. To assess whether effects of GY118F are dependent on STAT3, we introduced GY118F into Stat3 −/− and +/+ ES cells. This showed that only GY118F Stat3 +/+ ES cells could self-renew in N2B27 plus G-CSF ( Fig. 3a,b ). We can therefore conclude that GY118F action is dependent on STAT3 activation. However, we cannot exclude a potential contribution from JAK independent of STAT3. 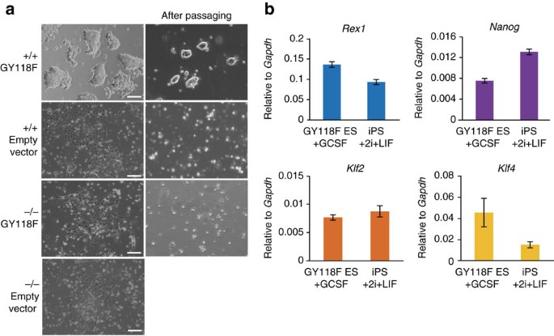Figure 3: The capacity of GY118F to sustain self-renewal is dependent on STAT3. (a) Phase images of GY118FStat3+/+andStat3−/−ES cells switched to N2B27 plus G-CSF. Empty vector transfectants were used as a control. White bars correspond to 123 μm. (b) qRT–PCR analysis of GY118FStat3+/+ES cells cultured in N2B27 plus G-CSF for pluripotency markers genes. Error bars indicate ±1 s.d. (n=3). Figure 3: The capacity of GY118F to sustain self-renewal is dependent on STAT3. ( a ) Phase images of GY118F Stat3 +/+ and Stat3 −/− ES cells switched to N2B27 plus G-CSF. Empty vector transfectants were used as a control. White bars correspond to 123 μm. ( b ) qRT–PCR analysis of GY118F Stat3 +/+ ES cells cultured in N2B27 plus G-CSF for pluripotency markers genes. Error bars indicate ±1 s.d. ( n =3). Full size image The ability of GY118F to enable reprogramming in N2B27 was also studied in female MEFs containing the Oct4-GFP reporter transgene. MEF pre-iPS generated by transduction of retroviral Oct4, Klf4, Sox2 and c-Myc, and subsequently transfected with GY118F gave rise to Oct4-GFP-positive colonies in N2B27 plus G-CSF ( Fig. 4a,b ). Subsequent characterization revealed a transcriptional profile characteristic of pluripotent cells, reactivation of the silent X-chromosome and dependency on continuous stimulation of the GY118F transgene ( Fig. 4c–g ). These cells could also be cultured interchangeably in 2i medium ( Fig. 4h ). 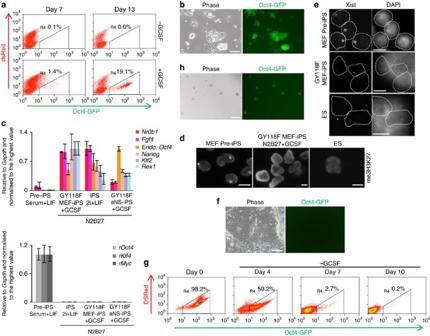Figure 4: GY118F enables reprogramming of mouse embryonic fibroblast-derived pre-iPS cells in N2B27. (a) Flow cytometry analysis of GY118F MEF-derived pre-iPS cells at day 7 and 13 after medium switch to N2B27 plus G-CSF. GFP expression indicates activation of the Oct4 reporter transgene. Percentage of Oct4-GFP-positive cells is indicated above the gate. (b) Phase and fluorescent images of GY118F Oct4-GFP-positive cells isolated and maintained in N2B27 plus G-CSF. The white bar corresponds to 151.2 μm. (c) qRT–PCR analysis for expression of pluripotency marker genes and retroviral (r) transgenes. iPS cells cultured in 2i plus LIF were used as a control. Gene expression and associated error bars, representing s.d. (n=3), were normalized to the sample with highest expression. Endo, endogenous. (d) Immunofluorescence of MEF-derived GY118F iPS cells for trymethyl(me3)H3K27. Pre-iPS cells and female ES cells were used as controls. White bars correspond to 19.6 μm. (e) FISH for Xist RNA on GY118F iPS cells. Pre-iPS cells were used as a control for presence of inactive X chromosome. Male ES cells were used as a positive control for Xist pinpoint signal. White dashed lines outline examples of individual cell nuclei. White bars correspond to 8.8 μm. (f) Phase and fluorescent images of GY118F iPS cells 9 days after withdrawal of G-CSF from N2B27. The white bar corresponds to 161.4 μm. (g) Flow cytometry analysis of GY118F iPS cells for Oct4-GFP expression on G-CSF withdrawal. Percentage of Oct4-GFP-positive cells is indicated above the gate. (h) Phase and fluorescent images of GY118F iPS cells after transfer to 2i medium. The white bar corresponds to 138.1 μm. Figure 4: GY118F enables reprogramming of mouse embryonic fibroblast-derived pre-iPS cells in N2B27. ( a ) Flow cytometry analysis of GY118F MEF-derived pre-iPS cells at day 7 and 13 after medium switch to N2B27 plus G-CSF. GFP expression indicates activation of the Oct4 reporter transgene. Percentage of Oct4-GFP-positive cells is indicated above the gate. ( b ) Phase and fluorescent images of GY118F Oct4-GFP-positive cells isolated and maintained in N2B27 plus G-CSF. The white bar corresponds to 151.2 μm. ( c ) qRT–PCR analysis for expression of pluripotency marker genes and retroviral (r) transgenes. iPS cells cultured in 2i plus LIF were used as a control. Gene expression and associated error bars, representing s.d. ( n =3), were normalized to the sample with highest expression. Endo, endogenous. ( d ) Immunofluorescence of MEF-derived GY118F iPS cells for trymethyl(me3)H3K27. Pre-iPS cells and female ES cells were used as controls. White bars correspond to 19.6 μm. ( e ) FISH for Xist RNA on GY118F iPS cells. Pre-iPS cells were used as a control for presence of inactive X chromosome. Male ES cells were used as a positive control for Xist pinpoint signal. White dashed lines outline examples of individual cell nuclei. White bars correspond to 8.8 μm. ( f ) Phase and fluorescent images of GY118F iPS cells 9 days after withdrawal of G-CSF from N2B27. The white bar corresponds to 161.4 μm. ( g ) Flow cytometry analysis of GY118F iPS cells for Oct4-GFP expression on G-CSF withdrawal. Percentage of Oct4-GFP-positive cells is indicated above the gate. ( h ) Phase and fluorescent images of GY118F iPS cells after transfer to 2i medium. The white bar corresponds to 138.1 μm. Full size image Taken together, these findings revealed that increased activation of JAK/STAT3 eliminates the requirement for additional pluripotency culture environment requisites in the promotion of somatic cell reprogramming to naïve pluripotency. JAK/STAT3 dominantly instructs naive pluripotency Increased activation of JAK/STAT3 was previously found to reprogramme EpiSCs to naïve pluripotency [8] . We stably transfected GY118F or empty vector into EpiSCs bearing an Oct4-GFP reporter. A comparison of GY118F-induced reprogramming efficiency in N2B27 alone to that supplemented with 2i plus LIF revealed that addition of 2i plus LIF enhances the efficiency of this process by only approximately twofold ( Fig. 5a ). The WT chimaeric LIF receptor was also shown to reprogramme EpiSCs when stimulated with G-CSF in combination with 2i plus LIF, but not in N2B27 only ( Fig. 5b,c ), demonstrating that this capacity is reliant on the Y118F mutation. For a transgene composed of STAT3 fused to the ligand-binding domain of the oestrogen receptor (STAT3ER), activation with tamoxifen led to reprogramming in N2B27 to which 2i and LIF were added, but not in N2B27 alone ( Fig. 5d ). It was previously shown that STAT3ER is not capable of inducing levels of Socs3 expression equivalent to those obtained with activated GY118F [8] . It is, therefore, likely that STAT3ER fails to reach a sufficient level of activity necessary to enable the induction of naïve pluripotency in N2B27 medium alone. 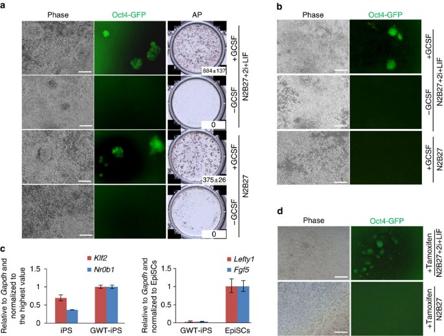Figure 5: JAK/STAT3 reprogrammes Epiblast stem cells to naive pluripotency in absence of further pluripotency culture requisites. (a) Phase and fluorescent images showing the emergence of Oct4-GFP-positive colonies (left and middle panels) and alkaline phosphatase (AP) staining (right panel) of GY118F EpiSCs reprogrammed in N2B27 or N2B27 plus 2i and LIF in the presence of G-CSF. Puromycin selection, which is under control ofOct4regulatory sequences, was used during 5 days prior AP staining to eliminate Oct4-GFP negative cells. AP staining was done in triplicate and a representative example is shown. The average colony number in N2B27 plus 2i plus LIF plus G-CSF was higher than for N2B27 Plus G-CSF (P=0.02 as determined byt-test). White bars correspond to 161.4 μm. (b) Reprogramming of EpiSCs containing a WT chimaeric LIF receptor, that is, that does not have the Y118F mutation. This shows emergence of Oct4-GFP-positive colonies in the presence of G-CSF in N2B27 plus 2i and LIF but not in N2B27 only. White bars correspond to 160.8 μm. (c) qRT–PCR analysis for naïve pluripotency and EpiSC marker genes of EpiSCs reprogrammed with the WT chimaeric LIF receptor (GWT) in 2i plus LIF medium. Gene expression and associated error bars representing s.d. (n=3) were normalized to the sample with highest expression. (d) STAT3ER reprogrammes EpiSCs in N2B27 plus 2i plus LIF, but not N2B27 alone, in the presence of tamoxifen. White bars correspond to 160.8 μm. Figure 5: JAK/STAT3 reprogrammes Epiblast stem cells to naive pluripotency in absence of further pluripotency culture requisites. ( a ) Phase and fluorescent images showing the emergence of Oct4-GFP-positive colonies (left and middle panels) and alkaline phosphatase (AP) staining (right panel) of GY118F EpiSCs reprogrammed in N2B27 or N2B27 plus 2i and LIF in the presence of G-CSF. Puromycin selection, which is under control of Oct4 regulatory sequences, was used during 5 days prior AP staining to eliminate Oct4-GFP negative cells. AP staining was done in triplicate and a representative example is shown. The average colony number in N2B27 plus 2i plus LIF plus G-CSF was higher than for N2B27 Plus G-CSF ( P =0.02 as determined by t -test). White bars correspond to 161.4 μm. ( b ) Reprogramming of EpiSCs containing a WT chimaeric LIF receptor, that is, that does not have the Y118F mutation. This shows emergence of Oct4-GFP-positive colonies in the presence of G-CSF in N2B27 plus 2i and LIF but not in N2B27 only. White bars correspond to 160.8 μm. ( c ) qRT–PCR analysis for naïve pluripotency and EpiSC marker genes of EpiSCs reprogrammed with the WT chimaeric LIF receptor (GWT) in 2i plus LIF medium. Gene expression and associated error bars representing s.d. ( n =3) were normalized to the sample with highest expression. ( d ) STAT3ER reprogrammes EpiSCs in N2B27 plus 2i plus LIF, but not N2B27 alone, in the presence of tamoxifen. White bars correspond to 160.8 μm. Full size image To identify downstream targets of GY118F, we performed microarray analysis on aNS-derived GY118F iPS cells that were reprogrammed and maintained in N2B27 plus G-CSF. These cells form a good assay system because they are completely and exclusively dependent on activation of GY118F to maintain pluripotency. G-CSF was withdrawn for 12 or 24 h so that genes that depend on JAK/STAT3 activation would be affected, but, at the same time, not long enough to induce differentiation. Subsequently, we re-added G-CSF to validate the response of these genes to GY118F. We chose to re-add G-CSF for the duration of 2 h and 40 min, because the response of known targets is clearly observed around this time. Genes of interest included those that were downregulated on withdrawal of G-CSF and upregulated on its re-addition and those with the converse gene expression pattern. The fold change in gene expression was required to be at least 1.4. Thirty-one genes met the criteria and thirteen of these had been previously reported as LIF/STAT3 downstream targets [23] , [24] , [25] ( Fig. 6a , GSE36818). Phosphorylated (p)-STAT3 levels dynamically responded to the withdrawal and re-addition of G-CSF, resulting in modulation of expression of downstream targets including Socs3 and Stat3 ( Fig. 6b ). The latter reflects STAT3's autoregulatory capacity. Klf4 , another known STAT3 target, met the applied fold-change criteria in all but the 12-h withdrawal microarray sample. This delay of Klf4 to respond to the lack of JAK/STAT3 activation could be explained by Klf4 also being positively regulated by the transcriptional network-controlling pluripotency. However, the trend for Klf4 was similar to that for Stat3 as confirmed by quantitative (q) RT–PCR analysis ( Fig. 6b ). Most of the putative downstream targets that had not previously been associated with JAK/STAT3 were verified by qRT–PCR in a biological replicate ( Supplementary Fig. S2 ). Transcriptional and protein levels of master pluripotency regulators Oct4 and Nanog were not affected ( Fig. 6c ), demonstrating both that the cells did not enter differentiation and that these are not part of the immediate mechanism by which GY118F induces pluripotency. In fact, Stat3 and Klf4 were the only two factors already known to promote induced pluripotency that were identified as GY118F downstream targets. 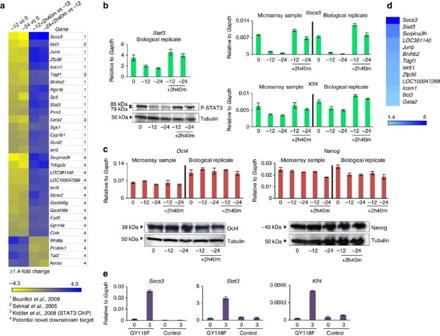Figure 6: Microarray analysis to identify GY118F downstream targets. (a–c). Experimental samples are GY118F iPS cells derived and maintained in N2B27 plus G-CSF (0), same cells but from which G-CSF was withdrawn for 12 or 24 h (−12, −24) and that subsequently had G-CSF added back for 2 h and 40 min (−12+2h40m, −24+2h40m). vs, versus. (a) Genes found by microarray array analysis that were either downregulated on G-CSF withdrawal and upregulated on re-addition of G-CSF or upregulated on G-CSF withdrawal and downregulated on re-addition of G-CSF. Yellow represents gene expression downregulation and blue upregulation. Range from −4.3- to +4.3-fold change, with a minimum of 1.4-fold change. (b) Western blot analysis for Phospho-STAT3 and qRT–PCR analysis for known JAK/STAT3 targetsStat3,Socs3andKlf4. Error bars indicate ±1s.d (n=3). (c) Western blot and q-RT–PCR analysis for pluripotency master regulators Oct4 and Nanog. Error bars indicate ±1 s.d. (n=3). (d) Genes that are upregulated in GY118F EpiSCs stimulated with G-CSF for 3 h, but not in controls, that were also found to be putative downstream targets of GY118F in iPS cells. (e) qRT–PCR analysis forSocs3,Stat3andKlf4in GY118F and control EpiSCs before (0), and after 3 h (3) of G-CSF stimulation. Error bars indicate ± 1 s.d (n=3). Figure 6: Microarray analysis to identify GY118F downstream targets. ( a – c ). Experimental samples are GY118F iPS cells derived and maintained in N2B27 plus G-CSF (0), same cells but from which G-CSF was withdrawn for 12 or 24 h (−12, −24) and that subsequently had G-CSF added back for 2 h and 40 min (−12+2h40m, −24+2h40m). vs, versus. ( a ) Genes found by microarray array analysis that were either downregulated on G-CSF withdrawal and upregulated on re-addition of G-CSF or upregulated on G-CSF withdrawal and downregulated on re-addition of G-CSF. Yellow represents gene expression downregulation and blue upregulation. Range from −4.3- to +4.3-fold change, with a minimum of 1.4-fold change. ( b ) Western blot analysis for Phospho-STAT3 and qRT–PCR analysis for known JAK/STAT3 targets Stat3 , Socs3 and Klf4 . Error bars indicate ±1s.d ( n =3). ( c ) Western blot and q-RT–PCR analysis for pluripotency master regulators Oct4 and Nanog. Error bars indicate ±1 s.d. ( n =3). ( d ) Genes that are upregulated in GY118F EpiSCs stimulated with G-CSF for 3 h, but not in controls, that were also found to be putative downstream targets of GY118F in iPS cells. ( e ) qRT–PCR analysis for Socs3 , Stat3 and Klf4 in GY118F and control EpiSCs before (0), and after 3 h (3) of G-CSF stimulation. Error bars indicate ± 1 s.d ( n =3). Full size image As a complementary cell system to further evaluate potential downstream targets identified in naïve pluripotent cells, we used EpiSCs. We performed microarray analysis for GY118F and control EpiSCs cultured in EpiSC medium supplemented with G-CSF for 3 h. We found that 48% of potential downstream targets positively regulated by GY118F in iPS cells were also upregulated in response to GY118F in EpiSCs ( P <0.01, >1.4-fold change) ( Fig. 6d , GSE36818). qRT–PCR analysis showed that activation of GY118F in EpiSCs induces expression of Klf4 (16-fold upregulation) ( Fig. 6e ). Stat3 expression levels increased by 11-fold, also a greater fold change than observed in naïve pluripotent cells ( Fig. 6e ). STAT3 is predicted to bind 73% of the identified GY118F targets common to both iPSCs and EpiSCs ( Supplementary Fig. S3 ). In accordance with the positive role of GY118F in induced pluripotency and self-renewal, most of its potential downstream targets in iPS cells were also previously found to be genomic binding targets of the pluripotency transcription factor network ( Supplementary Fig. S3 ). STAT3 and Klf4 are known to co-occupy genomic target sites with Oct4, Sox2 and Nanog, showing convergence of extrinsic signalling with the intrinsic core pluripotency circuitry [26] . As shown above, overactivation of JAK/STAT3 is sufficient to efficiently induce conversion of EpiSCs into naïve pluripotent cells in N2B27 alone. This prompted us to investigate whether a culture environment that adversely affects naïve pluripotency self-renewal could pose a barrier to GY118F-mediated reprogramming. In ES cells, FGF-ERK signalling triggers exit from self-renewal to enter lineage commitment [27] , [28] , [29] . This is in contrast to its effect on EpiSCs, which rely on FGF-ERK signalling that, together with, Activin promotes their self-renewal [30] . To address whether activation of FGF signalling blocks the ability of GY118F to induce naïve pluripotency, we attempted to reprogramme EpiSCs in N2B27 medium supplemented with both FGF and G-CSF. Despite the presence of FGF, Oct4-GFP-positive colonies emerged in cells where GY118F was activated ( Fig. 7a ). These stained positive for alkaline phosphatase ( Fig. 7a ) and could be serially passaged ( Fig. 7b ). Gene expression analysis showed both downregulation of EpiSC marker genes and upregulation of ES cell marker genes ( Fig. 7c ). Evaluation of the developmental potential of GY118F iPS cells derived and maintained in N2B27 plus FGF and G-CSF showed that these can contribute to chimaeras, confirming their naïve pluripotent state ( Fig. 7d ). 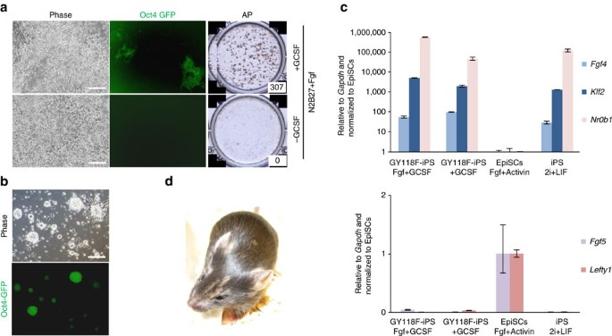Figure 7: Activation of JAK/STAT3 is dominant over FGF signalling for Epiblast stem cell reprogramming to naive pluripotency. (a–d) Reprogramming of GY118F EpiSCs in N2B27 plus FGF2 and G-CSF and subsequent analysis. (a) Phase and fluorescent images showing the emergence of Oct4-GFP-positive colonies and AP staining of GY118F cells. Puromycin selection was applied during 5 days prior AP staining to eliminate Oct4-GFP negative cells. White bars correspond to 161.4 μm. (b) Phase and fluorescent images of derived GY118F Oct4-GFP-positive cells maintained in N2B27 plus FGF plus G-CSF. White bars correspond to 161.4 μm. (c) qRT–PCR analysis for naïve pluripotency and EpiSC marker genes. An iPS cell line cultured in 2i plus LIF was used as a control for naïve pluripotent gene expression. Gene expression and associated error bars representing s.d. (n=3) were normalized to EpiSCs. (d) Agouti coat colour shows contribution of GY118F iPS cells derived and maintained in N2B27 plus FGF and G-CSF. Figure 7: Activation of JAK/STAT3 is dominant over FGF signalling for Epiblast stem cell reprogramming to naive pluripotency. ( a – d ) Reprogramming of GY118F EpiSCs in N2B27 plus FGF2 and G-CSF and subsequent analysis. ( a ) Phase and fluorescent images showing the emergence of Oct4-GFP-positive colonies and AP staining of GY118F cells. Puromycin selection was applied during 5 days prior AP staining to eliminate Oct4-GFP negative cells. White bars correspond to 161.4 μm. ( b ) Phase and fluorescent images of derived GY118F Oct4-GFP-positive cells maintained in N2B27 plus FGF plus G-CSF. White bars correspond to 161.4 μm. ( c ) qRT–PCR analysis for naïve pluripotency and EpiSC marker genes. An iPS cell line cultured in 2i plus LIF was used as a control for naïve pluripotent gene expression. Gene expression and associated error bars representing s.d. ( n =3) were normalized to EpiSCs. ( d ) Agouti coat colour shows contribution of GY118F iPS cells derived and maintained in N2B27 plus FGF and G-CSF. Full size image Derivation of EpiSCs and the self-renewal of these are attained by using N2B27 basal medium supplemented with FGF2 and Activin A [31] . If naïve pluripotent cells are cultured in this medium, they differentiate into an EpiSC state [31] . Direct reprogramming of somatic cells into an EpiSC-like state is also enabled by the use of Activin and FGF2 in the medium [5] . We therefore asked whether EpiSC culture conditions, which instruct and maintain the primed pluripotent state, would block JAK/STAT3 signalling from inducing naïve pluripotency. To investigate this, we used EpiSCs containing a GFP reporter transgene driven by regulatory sequences of Oct4 that include its distal enhancer but lack the proximal enhancer (ΔPE). This reporter is expressed in ES cells but silenced in EpiSCs [32] . Unexpectedly, on G-CSF stimulation of GY118F ΔPE EpiSCs, GFP-expressing colonies emerged within 1 week ( Fig. 8a ). By day 12 ~7% of the total number of cells activated the naïve pluripotency reporter ( Fig. 8b ). Because ΔPE Oct4-GFP expression was not coupled to an antibiotic resistance gene and the cells did not have a proliferative advantage over self-renewing EpiSCs, we isolated GFP-expressing cells by flow cytometry ( Fig. 8c ). Analysis of these showed that genes characteristic of naïve pluripotent cells were upregulated, whereas those expressed in EpiSC were downregulated ( Fig. 8d ). The obtained iPS cells could be interchangeably cultured in N2B27 supplemented with either G-CSF, 2i or Activin plus FGF plus G-CSF with or without inhibitors of Activin and Fgf signalling ( Fig. 8e ; Supplementary Fig. S4a ). The application and subsequent withdrawal of selective inhibitors of Fgf or Activin receptors, or the withdrawal and readdition of Activin and Fgf, led to a response of Activin and FGF target genes Lefty2 and Dusp4 , respectively ( Fig. 8f ). These data indicate that the obtained iPS cells are responsive to, but do not require Activin or Fgf signalling for self-renewal. In contrast, withdrawal of G-CSF resulted in loss of ΔPE Oct4-GFP expression ( Supplementary Fig. S4b ). Whereas, in female EpiSCs, one X chromosome is silenced, the reprogrammed cells exhibited loss of the Xist RNA cloud and appearance of Xist pinpoint signals indicative of X chromosome reactivation and acquisition of a naïve pluripotent cell state ( Fig. 8g ). Importantly, in contrast to EpiSCs [32] , GY118F iPS cells derived and maintained in EpiSC medium plus G-CSF were able to contribute to chimaeras on blastocyst injection ( Fig. 8h ). To ensure that the observed induction and stabilization of a naïve pluripotent state in EpiSC medium is not particular to the ΔPE EpiSCs, we investigated this capacity in an independent EpiSC line. We used TNGA EpiSCs that have a GFP reporter transgene under control of the regulatory sequences of the endogenous Nanog gene [33] . GFP expression from this reporter was undetectable in EpiSCs. However, on activation of GY118F in Activin and FGF culture conditions GFP-positive colonies emerged, which exhibited a gene expression profile characteristic of naïve pluripotency ( Supplementary Fig. S4c–e ). 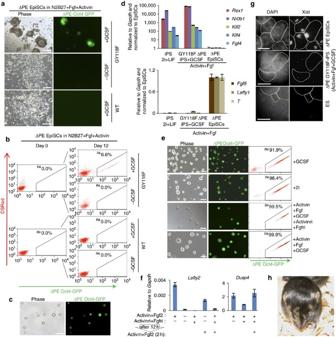Figure 8: JAK/STAT3 induces naive pluripotency despite a culture environment that instructs and maintains the primed cell state. (a–d) Reprogramming of GY118F ΔPE Oct4-GFP EpiSCs to naïve pluripotency in N2B27 plus Activin plus FGF plus G-CSF. (a) Phase and fluorescent images showing the emergence of ΔPE Oct4-GFP-positive colonies. White bars correspond to 161.4 μm. (b) Flow cytometry analysis of GY118F EpiSCs at day 0 and 12 days after the addition of G-CSF. Parental ΔPE EpiSCs were used as a negative control. The percentage of ΔPE Oct4-GFP-positive cells is indicated above the gate. (c) GY118F ΔPE Oct4-GFP-positive cells isolated and maintained in N2B27 plus Fgf2 plus Activin plus G-CSF. White bars correspond to 141.54 μm. (d) qRT–PCR analysis for naïve pluripotency and EpiSC marker genes. Gene expression and associated error bars representing s.d were normalized to EpiSCs. (e) Phase and fluorescent images of GY118F iPS cells derived and maintained in N2B27 with Activin plus Fgf plus G-CSF cultured with or without inhibitors for Activin (Activinri) and Fgf (Fgfri) signalling or cultured in N2B27 with 2i or G-CSF. White bars correspond to 143.9 μm. Flow cytometry analysis (right panel) confirming continued expression of the ΔPE Oct4-GFP reporter transgene in all culture conditions. (f) qRT–PCR analysis forLefty2andDusp4expression on addition and subsequent withdrawal of A8301 (Activinri) and PD173074 (Fgfri) inhibitors or withdrawal and readdition of Activin and Fgf from GY118F iPS cells. Error bars indicate ± 1 s.d (n=3). (g) FISH for Xist RNA on GY118F ΔPE Oct4-GFP iPS cells derived and maintained in Activin plus FGF plus G-CSF. ΔPE Oct4-GFP EpiSCs were used as a control for presence of an inactive X chromosome. Male ES cells were used as a positive control for presence of pinpoint signal. White dashed lines outline examples of individual cell nuclei. White bars correspond to 8.8 μm. (h) Contribution of GY118F ΔPE Oct4-GFP iPS cells derived and maintained in N2B27 plus Activin plus FGF plus G-CSF to chimaeras as reflected by agouti coat colour. Figure 8: JAK/STAT3 induces naive pluripotency despite a culture environment that instructs and maintains the primed cell state. ( a – d ) Reprogramming of GY118F ΔPE Oct4-GFP EpiSCs to naïve pluripotency in N2B27 plus Activin plus FGF plus G-CSF. ( a ) Phase and fluorescent images showing the emergence of ΔPE Oct4-GFP-positive colonies. White bars correspond to 161.4 μm. ( b ) Flow cytometry analysis of GY118F EpiSCs at day 0 and 12 days after the addition of G-CSF. Parental ΔPE EpiSCs were used as a negative control. The percentage of ΔPE Oct4-GFP-positive cells is indicated above the gate. ( c ) GY118F ΔPE Oct4-GFP-positive cells isolated and maintained in N2B27 plus Fgf2 plus Activin plus G-CSF. White bars correspond to 141.54 μm. ( d ) qRT–PCR analysis for naïve pluripotency and EpiSC marker genes. Gene expression and associated error bars representing s.d were normalized to EpiSCs. ( e ) Phase and fluorescent images of GY118F iPS cells derived and maintained in N2B27 with Activin plus Fgf plus G-CSF cultured with or without inhibitors for Activin (Activinri) and Fgf (Fgfri) signalling or cultured in N2B27 with 2i or G-CSF. White bars correspond to 143.9 μm. Flow cytometry analysis (right panel) confirming continued expression of the ΔPE Oct4-GFP reporter transgene in all culture conditions. ( f ) qRT–PCR analysis for Lefty2 and Dusp4 expression on addition and subsequent withdrawal of A8301 (Activinri) and PD173074 (Fgfri) inhibitors or withdrawal and readdition of Activin and Fgf from GY118F iPS cells. Error bars indicate ± 1 s.d ( n =3). ( g ) FISH for Xist RNA on GY118F ΔPE Oct4-GFP iPS cells derived and maintained in Activin plus FGF plus G-CSF. ΔPE Oct4-GFP EpiSCs were used as a control for presence of an inactive X chromosome. Male ES cells were used as a positive control for presence of pinpoint signal. White dashed lines outline examples of individual cell nuclei. White bars correspond to 8.8 μm. ( h ) Contribution of GY118F ΔPE Oct4-GFP iPS cells derived and maintained in N2B27 plus Activin plus FGF plus G-CSF to chimaeras as reflected by agouti coat colour. Full size image Together, these data show that increased JAK/STAT3 activation is a dominant cue that enforces naïve pluripotency despite a culture environment that otherwise instructs and stabilizes a primed state. This study attributes key properties to JAK/STAT3 that position it as one of the most potent reprogramming factors for the induction of naïve pluripotency. Increased JAK/STAT3 activation enabled reprogramming of somatic cells in the absence of additional pluripotency culture requisites and dominantly enforced naïve pluripotency in a culture environment that both instructs and maintains a primed state. The LIF receptor is already expressed in pre-iPS cells at levels two- to threefold higher than ES cells [14] . However, LIF alone cannot overcome the pre-iPS cell reprogramming block or instate pluripotency in N2B27 medium alone. One possibility could be that overexpression of the LIF receptor is all that is required. However, we did not observe reprogramming of EpiSCs in N2B27 medium alone using the WT chimaeric LIF receptor. The elimination of MEK/ERK and PI3-Kinase activation by the Y118F mutation may thus be beneficial for reprogramming, although neither FGF nor EGF (data not shown) stimulation blocked GY118F-mediated EpiSC conversion. The absence of negative feedback from Socs3 (refs 16 , 17 ), may be necessary for sufficient JAK/STAT3 activation to be reached. As a consequence of the negative feedback loop, p-STAT3 and Socs3 levels oscillate in opposite phase. Abolition of this feedback stops p-STAT3 oscillation and leads to persistent high levels of p-STAT3 (refs 16 , 34 ). Klf4 is a downstream target of JAK/STAT3 that is part of the transcriptional network governing pluripotency [35] . It is also one of the 'Takahashi & Yamanaka' reprogramming factors and is sufficient in 2i culture conditions to induce EpiSC reprogramming to naïve pluripotency [1] , [31] . Moreover, Klf4 overexpression can partially replace the requirement for LIF in ES cell self-renewal [36] . However, Klf4 cannot sustain self-renewal of ES cells in N2B27 alone or rescue Stat3 −/− ES cells [37] . In addition, Klf4 and LIF/STAT3 signalling are known to synergize to enhance reprogramming efficiency [8] . Interestingly, STAT3 and Klf4 are reported to co-occupy as much as 56.8 and 41.9%, respectively, of genomic multiple transcription factor binding loci bound by the core pluripotency transcription factors, thereby integrating signalling in the core transcriptional network [26] . In somatic cell reprogramming, JAK/STAT3 promotes induced pluripotency together with Oct4 and Klf4. In EpiSCs, Oct4 is already expressed and we showed that Klf4 expression can be induced by enforcing JAK/STAT3 signalling. Thus, cooperation of STAT3 and Klf4 with Oct4 may be an important driver to establish and maintain naïve pluripotency. Potential downstream mediators of JAK/STAT3 perform a variety of functions that could contribute to its reprogramming mechanism. Candidates include factors involved in cellular proliferation and inhibition of apoptosis, such as Pim3 and Bcl3. Pim3 has previously been shown to support ES cell self-renewal by reducing spontaneous differentiation and sensitivity to LIF starvation [38] . Apoptosis and cell cycle arrest were recently shown to comprise barriers for reprogramming [39] . In addition, JAK/STAT3 affects genes that may influence signalling like Tdgf1 and kinase Sgk1 that has been reported to phosphorylate GSK3 leading to its inactivation [40] . Inhibition of GSK3 is known to contribute to both naïve pluripotency self-renewal and reprogramming [4] , [21] . It is interesting to note that in a study where 24 STAT3 target genes were perturbed by short interfering RNA that 23 had an effect, although some only mildly, on the capacity of ES cells to maintain an undifferentiated state [23] . Although an increased understanding of the mechanism of JAK/STAT3 action will remain an interesting question for investigation, in a situation of conflicting signalling inputs, it seems that sufficiently elevated activation of JAK/STAT3 switches and locks the cell state into naive pluripotency. It is well known that mouse ES cells and current human ES cells lines, albeit exhibiting pluripotent characteristics, are different in particular in their signalling pathways governing pluripotency. Mouse EpiSCs have been shown to be remarkably similar in their signalling-pathway dependency to human ES cells [6] , [7] . Both human ES cells and mouse EpiSCs rely on FGF/MAPK and TGFβ/Activin/Nodal signalling pathways to sustain self-renewal [7] , whereas mouse ES cells rely on BMP4 and activation of LIF-STAT3 (ref. 20 ). EpiSCs exhibit in vitro differentiation capacity and have the ability to form teratomas. However, until today reports of EpiSCs re-entering embryonic development are limited. It is possible that human ES cells represent a population of cells that differ from mouse ES cells, because they correspond to a later time point in development or have adopted another non-naïve pluripotent state, rather than reflecting non-conserved properties between species. Culture conditions used for mouse somatic cell reprogramming and naïve ES cell maintenance have not been successful in supporting human ES cell derivation or reprogramming. It is possible that the identification of factors that make reprogramming less reliant on culture requirements may help capturing naïve pluripotent cells from non-rodent species, where the nature or even existence of culture conditions that support such a state are not known. The recent establishment of human ES cells with properties similar to mouse ES cells was achieved by constitutive expression of Klf4, together with Oct4 or Klf2, in combination with 2i and LIF culture conditions [41] . Interestingly, the obtained pluripotent cells were dependent on LIF signalling. It will be of interest to determine whether overactivation of JAK/STAT3 in human ES cells or somatic cells could lead to reprogramming into a cell state more akin to mouse naïve pluripotent cells. In conclusion, our studies demonstrated that sufficient levels of JAK/STAT3 activation exert a role as a master reprogramming factor that dominantly instructs naïve pluripotency. Plasmids GY118F and WT Chimaeric LIF receptor sequences are described in ref. 12 . To drive the expression of these, we used a PiggyBac vector containing both a CAG promoter driving the expression of dsRed and hygromycin resistance, linked by an IRES sequence, and a second CAG promoter driving GY118F or WT chimaeric LIF receptor expression. STAT3ER plasmid is described in ref. 23 . PMXs-Oct4, pMXs-Klf4, pMXs-cMycT58 and pMX Sox2 were obtained from Addgene repository. Cells PlatE cells were maintained in DMEM plus 10% serum in presence of puromycin and blasticydin selection. NS cells were maintained in RHBA (StemCells) supplemented with 10 ng ml −1 FGF2 (Home-made) and 10 ng ml −1 EGF (Peprotech) on gelatine-coated flasks. Pre-iPS cells were maintained on gelatin in GMEM (Gibco) supplemented with 10% fetal calf serum, pyruvate, glutamine, β-mercaptoethanol and non-essential amino acids. Mouse iPS cells were cultured as indicated in the text. N2B27 was made from DMEMF12 (Gibco) and Neurobasal (Gibco) in a 1:1 ratio supplemented with N2 (home-made or StemCells), B27 (Invitrogen), L -glutamine and β-mercaptoethanol. 2i medium was made by supplementing N2B27 with Chiron (3 μM), PDO3 (1 μM) and optionally with LIF. IPS cells were grown on either gelatin or Poly- L -ornithine hydrobromide plus Laminin- (from Engelbreth-Holm-Swarm murine sarcoma basement membrane) coated plates or flasks. EpiSCs were maintained in N2B27 plus 20 ng ml −1 Activin and 12.5 ng ml −1 FGF2 on fibronectin-coated plates or flasks. Murine recombinant G-CSF was purchased from Peprotech and used at a concentration of 30 ng ml −1 . A8301 was used at a concentration of 1 μM. PD173074 was used at a concentration of 0.1 μM. Transfection of PiggyBac vector into NS and pre-iPS cell lines was performed by nucleofection of plasmid DNA with the Lonza (amaxa) cell nucleofector, protocol T-020 (kit V). Transfection of PiggyBac vector into EpiSCs was made by lipofection (Invitrogen lipofectamine 2000). For Piggybac vectors, 1 μg plasmid plus 2 μg pBase transposase was used. Retroviral infection and reprogramming assays Plat-E cells were seeded at 2×10 6 cells per 10 cm ø dish. The following day Plat-E cells were transfected with 9 μg of either PMX retroviral Oct4, Klf4, c-Myc or Sox2 with FuGENE 6 transfection reagent (Roche). The next day, plat-E medium was replaced and 1.2×10 5 MEFs or NS cells per 10 cm 2 well were plated. After 24 h, Plat-E supernatants were filtered, enriched with 4 μg ml −1 polybrene (Sigma-Aldrich) and mixed. The target cells where incubated with this supernantant for 24 h. Sox2 was only included for MEF infection. Then medium was subsequently changed accordingly to MEFs or NS cell culture requirements. For MEFs on the emergence of pre-iPS cells, clonal lines were derived. For pre-iPS cell reprogramming, 6×10 4 or 1×10 5 cells were plated per 10 cm 2 and switched to the experimental culture conditions 48 h later. EpiSCs were plated at 2×10 4 to 8×10 4 cells per 10 cm 2 well and switched to the experimental culture conditions within 1–4 days. Alkaline phosphatase staining Cells were fixed in citrate-acetone-formaldehyde and subsequently stained for alkaline phosphatase with the alkaline phosphatase-staining leukocyte kit (Sigma-Aldrich) according to manufacturer's recommendations. Quantitative real-time PCR RNA was isolated using RNeasy kit (Qiagen) and reverse transcribed into complementary DNA using superscriptIII (Invitrogen). qRT–PCR was accomplished using Taqman probes with Taqman fast universal PCR master mix (Applied Biosystems) or gene-specific primers with SYBR green (Applied Biosystems). The full list of probes and primers used can be found in the Supplementary Tables S1–S3 . qRT–PCR experiments were performed on the 7900 HT Fast Real-Time PCR System or StepOnePlus Real-Time PCR System (Applied Biosystems). For taqman qRT–PCR, average threshold cycles were determined from triplicate reactions and the levels of gene expression were normalized to GAPDH (VIC-labelled endogenous control assay). Error bars indicate ±1 standard deviation or standard deviation normalized to a reference sample, as indicated in the legend. For SYBR green qRT–PCR, mean quantity of expression was determined from triplicate reactions and a standard curve. Expression levels were normalized to GAPDH . Error bars indicate ±1 standard deviation. Immunohistochemistry Cells were plated on glass slides and permiabilized with 0.3%. triton PBS for 4 min, before fixation in 4% PFA for 20 min. Polyclonal antibody to trimethyl H3-K27 from Upstate was used at a concentration of 1 in 500. Chimaeras iPS cells from a 129xMF1 (Oct4-GFP) or 129 (ΔPEOct4-GFP) origin were microinjected in C57BL/6 host blastocysts. Contribution of the injected iPS cells is reflected by agouti coat colour. Microarray Microarrays were performed on the Illumina MouseWG-6 v2.0 Expression BeadChips. The data were loaded into the R package lumi [42] . A given probe needed to abide to the Illumina detection p-value of 0.01 in at least one of the samples. If failing, this probe was excluded from analysis to prevent noise. Subsequently, the data was transformed using variance stabilization [43] and then normalized using quantile normalization. The samples analysed were GY118F iPS cells in N2B27 plus G-CSF (t0), same cells but from which G-CSF was withdrawn for 12 or 24 h ( t -12, t -24) and to which subsequently G-CSF was added back for 2 h and 40 min ( t -12+2 h40m, t -24+2 h40m). Samples t -12 and t -24 were compared to t 0. Samples t -12+2 h40m and t -24+2 h40m were compared to t -12 and t -24, respectively. For the microarray performed for GY118F and Control EpiSCs in EpiSC medium, GY118F and control-EpiSCs before G-CSF stimulation (triplicate samples), and Control EpiSCs after 3 h of G-CSF stimulation (triplicate samples) and GY118F EpiSCs after 3 h of G-CSF stimulation (duplicate samples) were analysed. Genes of interest were defined as those that were significantly upregulated ( P <0.01) above a defined threshold in G-CSF-stimulated GY118F EpiSCs as compared with those not stimulated, but for which the expression did not significantly change on G-CSF stimulation in the control. The fold change in expression was calculated by 2^absolute value of subtracted normalized data. The microarray data have been deposited in the GEO database under accession code GSE36818 . Western blotting Mouse monoclonal α-tubulin antibody (Santa Cruz Biotechnology) was used at a concentration of 1 in 5,000 and rabbit polyclonal antibodies to phospho-STAT3, STAT3, phospho-Erk and total ERK (Cell Signaling) were used at 1 in 1,000. Mouse monoclonal Oct4 antibody (Santa Cruz) and rat monoclonal nanog antibody (eBioscience) were used at 1 in 500. RNA Fluorescent in situ hybridization Cells were permeabilized in cytoskeletal buffer (100 mM NaCl, 300 mM sucrose, 3 mM MgCl2, 10 mM PIPES) containing 0.5% Triton X-100, 1 mM EGTA pH 8 and vanadyl ribonucleoside (New England Biolabs), for 5 min. They were subsequently fixed in 4% paraformaldehyde for 10 min, briefly washed in PBS and dehydrated through 70, 80, 95 and 100% ethanol, after which the slides were air-dried. At this stage, a denatured Xist probe was applied onto the slide and these were incubated overnight at 37 °C. The probe was prepared by labelling plasmid DNA containing a mouse Xist exon 1 fragment sequence (gift from Professor Neil Brockdorff) with a biotin-nick translation mix (Roche) according to manufacturer's instructions and removing non-incorporated nucleotides with an S-300HR Illustra microspin column (GE Healthcare). To 20 ng of probe, 10 μg of sheared salmon sperm DNA (Ambion) and 3 μg of mouse Cot-1 DNA (Invitrogen) was added. Finally, the probe was dehydrated, resuspended in deionized formamide, denatured at 80 °C, added to 2× hybridization buffer (4xSSC, 20% dextran sulphate, 2 mg ml −1 BSA, 2 mM vanadyl ribonucleoside) and applied to the slide. The following day, the slides were washed in 2xSSC/50% formamide for 15 min, then 3 times in 2xSSC, transferred to 4xSSC/0.1% Tween20 and finally blocked in 4xSSC, 0.1%Tween20, 4 mg ml −1 BSA. Probe detection was performed by first applying Avidin conjugated to Texas Red (1/500, Vector Laboratories), then a biotinylated anti-avidin antibody (1/200, Vector Laboratories), followed by a second layer of Avidin-Texas Red. All detection reagents were diluted in 4xSSC, 0.1% Tween20, 1 mg ml −1 BSA and incubated at 37 °C for 30 min followed by three washes in 4xSSC/0.1% Tween20 in between each step. Finally, the slides were mounted in Vectashield Mounting Medium containing DAPI (Vector Laboratories). Analysis of putative transcription factor binding Putative binding was predicted from consideration of publicly available ChIP-seq data. Studies included were: GSE11431_Stat3, GSE11431_Klf4, GSE11431_Esrrb, GSE11431_Oct4, GSE11724_Oct4, GSE22934_Oct4, GSE11724_Sox2, GSE11431_Sox2, GSE11431_Nanog, GSE11724_Nanog. Raw ChIP-seq data sets for selected transcription factors in ES cells were downloaded from the Gene Expression Omnibus (GEO, http://www.ncbi.nlm.nih.gov/geo/ ), realigned to the mouse genome (mm9) with the bowtie software ( http://bowtie-bio.sourceforge.net ), and peaks were called with MACS software ( http://liulab.dfci.harvard.edu/MACS ) using default parameters. For each gene, the transcription factor ChIP-seq peaks upstream (up to 20 kb) of the transcription start site, in the genic region, or downstream (2 kb) of the gene end, were determined. If at least one of the included studies for each considered transcription factor showed significant binding, this transcription factor was depicted in the graph to bind. Accession codes: The microarray data have been deposited in the GEO database under accession code GSE36818 . How to cite this article: van Oosten, A.L. et al . JAK/STAT3 signalling is sufficient and dominant over antagonistic cues for the establishment of naïve pluripotency. Nat. Commun. 3:817 doi: 10.1038/ncomms1822 (2012).